The discovery of kimberlites in Antarctica extends the vast Gondwanan Cretaceous province Kimberlites are a volumetrically minor component of the Earth’s volcanic record, but are very important as the major commercial source of diamonds and as the deepest samples of the Earth’s mantle. They were predominantly emplaced from ≈2,100 Ma to ≈10 ka ago, into ancient, stable regions of continental crust (cratons), but are also known from continental rifts and mobile belts. Kimberlites have been reported from almost all major cratons on all continents except for Antarctica. Here we report the first bona fide Antarctic kimberlite occurrence, from the northern Prince Charles Mountains, emplaced during the reactivation of the Lambert Graben associated with rifting of India from Australia-Antarctica. The samples are texturally, mineralogically and geochemically typical of Group I kimberlites from more classical localities. Their ≈ 120 Ma ages overlap with those of many kimberlites from other world-wide localities, extending a vast Cretaceous, Gondwanan kimberlite province, for the first time, into Antarctica. Kimberlites are rare, highly silica-undersaturated, mantle-derived igneous rocks, which have been emplaced into the crust, particularly in ancient and geologically stable cratons. Their trace element enrichments, small volumes, low silica but highly magnesian and volatile (C–H–O)-rich character argue that they represent melt compositions formed in the presence of H 2 O and CO 2 , very close to the carbonate–peridotite solidus [1] , [2] , [3] . The occasional but scientifically and commercially highly significant presence of diamonds suggests that they originated by partial melting of the mantle at extreme depths (>150 km), and some kimberlites (that is, those transporting diamonds with inclusions representing rare transition zone and lower mantle mineral phases) are the most deeply derived materials accessible on Earth. Kimberlites were emplaced over a significant period of geological history, ranging in age from the Palaeoproterozoic to the Cenozoic Eras, and have been reported on all continents except Antarctica [4] , [5] . Here we present mineralogical and geochemical data from three new kimberlite samples obtained from the southeastern slopes of Mt Meredith in the northern Prince Charles Mountains (nPCM) of Antarctica. These rocks represent the first reported occurrence of genuine kimberlite in Antarctica. Sample locations and petrography and mineralogy The location from which the samples were recovered is shown in Fig. 1 . One sample (77063) was obtained in situ from an outcrop, and the others (77081 and 77082) were recovered from boulders in till several metres from the outcrop. The three samples are classified as Group I kimberlites on the basis of petrography and mineral chemistry. They are strongly porphyritic with rounded to euhedral olivine crystals up to several millimetres across and rare phlogopite macrocrysts in a very fine-grained groundmass. Olivine crystals are partially replaced by serpentine on rims and along fractures ( Fig. 2a, b ), but all samples retain abundant fresh olivine. Most olivine crystals are rounded to euhedral in shape and up to 200 μm across. Others are larger (>1 mm across) and irregular in shape, and sometimes contain inclusions of phlogopite, orthopyroxene, Cr-diopside-rich clinopyroxene, perovskite and Cr-spinel ( Fig. 2c ). Olivine crystals vary significantly in major and minor element compositions (from Fo 74 to Fo 91 ; 0.02–0.45 wt% NiO and 0.10–0.50 wt% CaO). In some cases, they are interpreted as xenocrysts of lithospheric material rather than as phenocrysts. For example, one large olivine crystal has an embayed and resorbed core of Fo 90.5 olivine overgrown by a thin rim of Fo 88 olivine. The core contains separate inclusions of Cr- and Na-rich clinopyroxene as well as low Al and Ca orthopyroxene, which are compositionally similar to peridotitic phases from the upper mantle. Phlogopite macrocrysts can be up to several millimetres in length and are irregular to tabular in shape. Phlogopite Mg # [100*Mg/(Mg+∑Fe)] varies from 87.3 to 93.4. 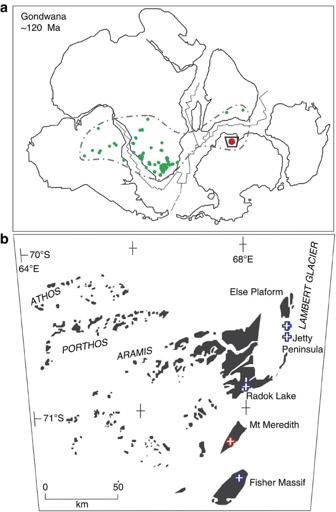Figure 1: Localities of 120 Ma old Gondwanan kimberlites. (a) Reconstruction of Gondwana at ~120 Ma (adapted from Veeverset al.40). The nPCM kimberlite occurrence is marked as a red dot. Other Cretaceous Gondwanan kimberlites5,27,30,31,32,33,41,42are shown as smaller green dots surrounded by a dashed line, broadly defining a vast Gondwanan, Cretaceous kimberlite province, which is extended into Antarctica by the newly discovered nPCM kimberlites; (b) Enlargement of the area surrounding the nPCM kimberlite localities, showing the location of samples 77063, 77081 and 77082 from Mt Meredith (red/white cross). When combined with the locations of nearby Cretaceous alkaline ultramafic and mafic rocks and carbonatites9,10,15(blue/white crosses), they form a linear feature parallel to the Lambert Graben, in which the Lambert Glacier flows. The length of the scale bar inbis 50 km. Representative mineral compositions are presented in Table 1 Figure 1: Localities of 120 Ma old Gondwanan kimberlites. ( a ) Reconstruction of Gondwana at ~120 Ma (adapted from Veevers et al. [40] ). The nPCM kimberlite occurrence is marked as a red dot. Other Cretaceous Gondwanan kimberlites [5] , [27] , [30] , [31] , [32] , [33] , [41] , [42] are shown as smaller green dots surrounded by a dashed line, broadly defining a vast Gondwanan, Cretaceous kimberlite province, which is extended into Antarctica by the newly discovered nPCM kimberlites; ( b ) Enlargement of the area surrounding the nPCM kimberlite localities, showing the location of samples 77063, 77081 and 77082 from Mt Meredith (red/white cross). When combined with the locations of nearby Cretaceous alkaline ultramafic and mafic rocks and carbonatites [9] , [10] , [15] (blue/white crosses), they form a linear feature parallel to the Lambert Graben, in which the Lambert Glacier flows. The length of the scale bar in b is 50 km. 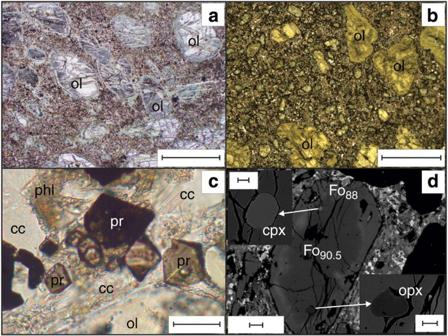Figure 2: Petrographic features of the Antarctic kimberlites. (a–c) Plain light photomicrographs of the Antarctic kimberlites (a,bandc– samples 77081, 77063 and 77082, respectively) showing porphyritic texture and olivine alignment. Olivine (ol) crystals are set in a fine- to coarse-grained groundmass, consisting of phlogopite (phl), calcite (cc), perovskite (pr), apatite and magnetite. Scale bar is 2 mm long inaandband 20 μm long inc. (d) Backscattered electron image of zoned olivine crystal with euhedral inclusions of high-Ca (cpx; upper left insert) and low-Ca (opx; lower right insert) pyroxenes in the resorbed core (sample 77082). Scale bar is 100 μm long in the main panel, 10 μm long in the upper left insert and 30 μm long in the lower right insert. Full size image Figure 2: Petrographic features of the Antarctic kimberlites. ( a – c ) Plain light photomicrographs of the Antarctic kimberlites ( a , b and c – samples 77081, 77063 and 77082, respectively) showing porphyritic texture and olivine alignment. Olivine (ol) crystals are set in a fine- to coarse-grained groundmass, consisting of phlogopite (phl), calcite (cc), perovskite (pr), apatite and magnetite. Scale bar is 2 mm long in a and b and 20 μm long in c . ( d ) Backscattered electron image of zoned olivine crystal with euhedral inclusions of high-Ca (cpx; upper left insert) and low-Ca (opx; lower right insert) pyroxenes in the resorbed core (sample 77082). Scale bar is 100 μm long in the main panel, 10 μm long in the upper left insert and 30 μm long in the lower right insert. Full size image Table 1 Representative electronprobe microanalyzer analyses of phases in the three samples. Full size table The fine-grained groundmass is mainly composed of calcite, olivine, phlogopite, magnesiochromite, Ti-magnetite, perovskite and apatite ( Fig. 2c ). Spinel exhibits distinctive atoll structures, in which euhedral cores of compositionally zoned magnesiochromite are surrounded by concentrically arranged zones of silicate material, which are in turn surrounded by magnetite. Very similar atoll spinels have been reported in other kimberlites [6] . Perovskite crystals are up to 100 μm across and perfectly octahedral ( Fig. 2c ). They formed in the groundmass and are also included in some olivine rims. Abundant anhedral calcite crystallized interstitially to other groundmass phases and makes up 10–12 modal% of the rocks. The association of xenocrystic and phenocrystic olivine and phlogopite macrocrysts set in a matrix containing perovskite, spinel, apatite and carbonate is a distinctive feature of kimberlites [4] , [7] . Notably, clinopyroxene does not occur as phenocrysts nor in the groundmass, precluding classification of these samples as ultramafic lamprophyres (UML) [8] , examples of which have been reported from other localities in the nPCM region [9] , [10] , [11] , [12] . Whole rock geochemistry The rocks are ultrabasic (29.2 to 32.1 wt% SiO 2 ) and have high MgO (19.1–27.3 wt%), CaO (10.9–28.8 wt%), CaO/Al 2 O 3 (2.7–2.9) and CO 2 (5.3–9.0 wt%), but low Al 2 O 3 contents (3.8–6.5 wt%), reflecting the observed olivine- and calcite-rich mineralogy. Large ranges in K 2 O (1.3–2.8 wt%) and P 2 O 5 (0.59–0.89 wt%) contents mainly reflect varying modal abundances of phlogopite and apatite, respectively. Na 2 O contents are very low (<0.15 wt%). On a plot of bulk SiO 2 /MgO versus MgO/CaO ( Fig. 3a ), the samples lie within a field of representative kimberlites [6] . Mesozoic UML from nearby Beaver Lake [12] have higher SiO 2 /MgO values (≥2) and are mostly outside the kimberlite field. 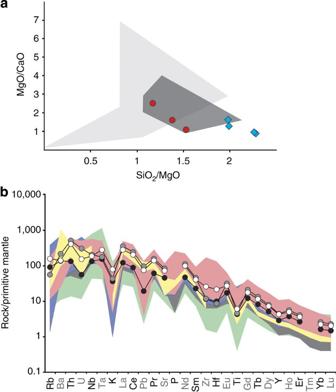Figure 3: Whole rock geochemical characteristics of the Antarctic kimberlites. (a) Plot of whole-rock SiO2/MgO versus MgO/CaO for the samples 77081, 77063 and 77082 (red dots) compared with Mitchell’s6field for representative, average kimberlites (dark grey shading), for extreme kimberlite compositions (light grey shading) and the UML from nearby Beaver Lake (Jetty Peninsula)12(blue diamonds). (b) Primitive-mantle normalized13, extended trace element plot of the three nPCM kimberlites (77081, black circles; 77063, white circles; and 77082, grey circles) compared with the range of values from a representative suite of 167 kimberlites from Africa (pink), Canada (yellow), Greenland (grey), India (indigo) and Siberia (green)43,44,45,46,47,48,49,50,51. Figure 3: Whole rock geochemical characteristics of the Antarctic kimberlites. ( a ) Plot of whole-rock SiO 2 /MgO versus MgO/CaO for the samples 77081, 77063 and 77082 (red dots) compared with Mitchell’s [6] field for representative, average kimberlites (dark grey shading), for extreme kimberlite compositions (light grey shading) and the UML from nearby Beaver Lake (Jetty Peninsula) [12] (blue diamonds). ( b ) Primitive-mantle normalized [13] , extended trace element plot of the three nPCM kimberlites (77081, black circles; 77063, white circles; and 77082, grey circles) compared with the range of values from a representative suite of 167 kimberlites from Africa (pink), Canada (yellow), Greenland (grey), India (indigo) and Siberia (green) [43] , [44] , [45] , [46] , [47] , [48] , [49] , [50] , [51] . Full size image Incompatible trace element concentrations tend to be high (generally >100 × Primitive Mantle [13] or more). For example, Rare Earth Element (REE) patterns are strongly light REE-enriched ([La/Yb] n =74–136), similar to kimberlites from other continents. K, Pb, Zr, Hf and Ti are depleted relative to trace elements of similar incompatibility (La, Ce, Sm, Eu and Gd) ( Fig. 3b ). The abundances of all measured incompatible trace elements and the general form of the Primitive Mantle normalized patterns match very closely kimberlites from other world-wide localities ( Fig. 3b ). Full whole rock analyses for the current samples are reported in Table 2 . Table 2 Whole rock major and minor element analyses determined by XRF and trace element analyses determined by ICP-MS. Full size table Radiometric ages of the samples Perovskite U–Pb dating by the laser ablation inductively coupled plasma mass spectrometry (LA-ICP-MS) method yielded apparent ages of 113±13 Ma (2 σ ) (77063), 125±8 Ma (77081) and 121±13 Ma (77082, see Methods section U–Pb LA-ICP-MS dating of perovskite). Assuming the perovskites are coeval, we obtain a weighted age of 122±6 Ma. This is supported by a 117±1 Ma Rb–Sr age for phlogopite from 77063 ( Table 4 ). On the basis of these ages, it is likely that that samples 77081 and 77082, from boulders within till are related in terms of age, to the kimberlite from which 77063 was sampled. An origin from the same kimberlite pipe, however, is unlikely given the diversity in initial Sr, Nd, Hf and Pb isotope ratios ( 87 Sr/ 86 Sr 0.7042−0.7054, ε Nd +1.9 to −2.1, ε Hf +4.6 to −5.5, 206 Pb/ 204 Pb 18.04−18.42, see Tables 3 , 4 , 5 ). The bulk rock 87 Sr/ 86 Sr for 77063 (0.7054±1) is supported by in situ Sr isotope data for perovskite (0.70539±12, see Supplementary Fig. S1 ). These radiogenic isotope signatures are intermediate between those established for Group I and transitional kimberlites from southern Africa [14] . Table 4 Rb–Sr dating of 77063 PHLOG. Full size table Table 3 Rb–Sr and Sm–Nd isotope results. Full size table Table 5 Lu–Hf and U–Pb isotope results. Full size table Ultramafic–mafic alkaline, carbonatitic and kimberlite-like rocks of similar age have been reported from elsewhere in the nPCM region, including Else Platform, Radok Lake and on the Fischer Massif, adjacent to the Lambert rift [9] , [10] , [15] . These rocks were classified as UML (alnöites), alkaline picrites, ultrabasic foidites, trachybasalts and carbonatite–kimberlites. In particular, Egorov et al. [16] reported the ‘first Antarctic occurrence of a dike kimberlite’ in the nPCM, inferred to be Early Cretaceous in age. However, samples from this dyke are significantly different from the current samples in that olivine macrocrysts (containing mantle-derived clinopyroxene and orthopyroxene inclusions – Fig. 2d ), garnet xenocrysts, ilmenite and perovskite are not reported. However, globular ‘syngenetic calcite carbonatite schlieren’ were present. In addition, the dyke is compositionally outside the range for kimberlites with low MgO (17 wt%) and Ni (480 ppm), reflecting the low modal olivine. We argue that this dyke is not a bona fide kimberlite, but more akin to a carbonatite magma that fractionated into a calcite-rich component and an apatite+magnetite+olivine component. The bona fide kimberlites described here and the other nPCM ultrabasic rock correlates appear to define a N–S linear feature extending 150 km along the margin of the Lambert rift ( Fig. 1b ). Interestingly, the UML occur in the northern part of the region (mainly around Beaver Lake) [9] , [10] , [11] , [12] , whereas the current kimberlites and the carbonatite–kimberlite reported by Belyatsky et al. [15] occur in the southern part. This may reflect progressive stages of development of the Lambert rift, with the UML representing a greater extent of rifting in the north, more erosion of the base of the lithosphere leading to melting at shallower subcontinental lithospheric levels, relative to the kimberlites in the south. Similar models have been suggested in the Ailik Bay rift [17] , and in the currently active rift in the western branch of the East African Rift system [18] . Kimberlites and related alkaline igneous rocks occur in all major Gondwanan continents (Africa, India, South America and Australia), but have not previously been reported from Antarctica. Kimberlite emplacement ages show well-developed clustering throughout the Mesoproterozoic, early Paleozoic, Mesozoic and Cenozoic [5] . In the Mesozoic, major emplacement events occurred 240, 145, 120, 85 and 73 Ma ago. The ca . 120 Ma episode was distributed particularly widely across the Gondwanan continents, and discovery of 120 Ma kimberlites in East Antarctica further extends this vast Cretaceous kimberlite province ( Fig. 1a ). At 120 Ma India and amalgamated Antarctica-Australia had already begun to drift apart, with early sea-floor spreading forming the proto-Indian Ocean [19] . The graben, on the margin of which the current kimberlites were emplaced, is a 700 km long zone of thinned continental crust believed to represent either a failed, trans-tensional basin that was activated 120 Ma ago during early extension associated with break-up of India and Antarctica-Australia [20] , [21] , or an accommodation zone related to a Carboniferous-Permian intracontinental rift between India and Antarctica, which was reactivated in the Cretaceous during continental dispersion [22] . Whichever the case, the nPCM kimberlites (and related alkali rocks of similar age at nearby locations [10] , [12] , [15] – Fig. 1 ) are most likely a magmatic expression of reactivation of pre-existing lithospheric discontinuities associated with the Lambert Graben during opening of the proto-Indian ocean. Kent [23] reported orangeites of age 109–116 Ma peripheral to the Bay of Bengal, India (Damodar Valley), which may relate to the same Cretaceous kimberlite province. Jelsma et al. [5] have shown that the time intervals in which kimberlite emplacement events were concentrated, coincided with fundamental plate reorganizations, such as supercontinent break-up. Thus, as well as constituting the first-known bona fide Antarctic kimberlite occurrence, the location of the nPCM kimberlites is consistent with models relating kimberlite distribution to reactivation of major trans-lithospheric structures during continental scale tectonic events [5] , and likely marks the onset of the reactivation of continental rifting zones, that is, similar to suggestions for other rift-related continental mantle-derived magmas such as carbonatites, UML and kamafugites (this study and refs 17 , 18 ). Thus, the Antarctic kimberlites and previously reported UML as well as other alkaline volcanics in the nPCM region potentially provide rare insights into large-scale tectonic mantle processes during the Cretaceous. Electronprobe microanalysis Constituent mineral phases in the samples were analysed for major and minor elements using a Cameca SX-50 WDS electronprobe microanalyser at Macquarie University. The accelerating voltage was 15 kV and beam current was 20 nA. Count times varied from 20 s on major elements to 60 s on minor elements. Calibration was performed on natural mineral standards. Representative data is presented in Table 1 . X-ray fluorescence analysis Whole rock major and minor element abundances were determined on powdered samples using X-ray fluorescence (XRF) microscopy, at Macquarie University ( Table 2 ). Solution – ICP-MS analysis Trace element abundances in the chilled margins were measured by solution – ICP-MS at the Australian National University (ANU) following procedures similar to those described by Norman et al. [24] ( Table 2 ). Isotopic analyses Rb–Sr and Sm–Nd isotope analyses were performed on leachate–residue pairs. Sample 77063 (105 mg, fine crush) was leached with cold 2M HCl (12 h), whereas rock powders for 77081A and 77082A were leached with cold 6M HCl. After removal of the clear solution, the residues were dried and re-weighed to determine weight loss during acid leaching. The residues were dissolved at low pressure using HF/HNO 3 and HCl. Following preliminary semi-quantitative trace element analysis, all fractions were spiked with 85 Rb– 84 Sr and 149 Sm– 150 Nd tracers, followed by extraction of Rb, Sr and LREE using conventional cation exchange and EICHROM Sr and LN resins [25] . Total analytical blanks (<0.1 ng) were negligible. Isotopic analyses were carried out on a NU Plasma multi-collector ICP-MS coupled to a CETAC Aridus desolvator. As part of an online iterative spike removal/mass bias correction procedure, instrumental mass bias was corrected by internal normalization to 88 Sr/ 86 Sr=8.37521 and 146 Nd/ 145 Nd=2.0719425 (equivalent to 146 Nd/ 144 Nd=0.7219 (ref. 26 )); data are reported relative to SRM987=0.710230 and La Jolla Nd=0.511860. Typical in-run precisions (two standard errors) are ±0.000020 (Sr) and ≤±0.000010 (Nd), whereas external (2 σ ) precisions – based on rock standards – are ±0.000020 (Nd) and ±0.000040 (Sr). External precision (2 σ ) for 87 Rb/ 86 Sr and 147 Sm/ 144 Nd is ±0.5% and ±0.2%, respectively. 147 Sm/ 144 Nd and 143 Nd/ 144 Nd in modern CHUR is 0.1967 and 0.512638. Initial 87 Sr/ 86 Sr(t) and ε Nd (t) were calculated for t =120 Ma. Results for standards (±2 s.d.) are as follows: BCR-2 ( n =2); Rb 46.8 ppm, Sr 339 ppm, 87 Rb/ 86 Sr 0.400, 87 Sr/ 86 Sr 0.70502, Sm 6.48 ppm, Nd 28.32 ppm, 147 Sm/ 144 Nd 0.1382, 143 Nd/ 144 Nd 0.512629; 0.512640±17 (mean of 21 runs of BCR-2 in 2010), 0.705015±34 (mean of 8 runs of BCR-2 in 2010–2011: JNd-1; 0.512114±23 (mean of 9 runs in 2010); BHVO-2 0.512992±17 (mean of 6 runs in 2010). Results are consistent with Thermal Ionisation Mass Spectrometry (TIMS) reference values. Uncertainties in initial ratios are: 87 Sr/ 86 Sr ±0.00010; ε Nd ±0.5 units. The decay constants are: 87 Rb 1.42 10 −11 /yr, 147 Sm 6.54 10 −12 /yr. Rb–Sr dating of megacrystic phlogopite from sample 77063 was done on euhedral (1–3 mm) mineral flakes. Two handpicked fractions (2–4 mg) were cleaned in 0.1M HNO 3 , spiked with 87 Rb– 84 Sr tracer and dissolved on a hotplate. Sr was extracted and purified using two passes over a small (0.1 ml) column of EICHROM Sr-resin (50–100 μm). Rb was extracted using cation resin chromatography (4 ml of AG50-X8, 200–400 mesh). Sr isotope data were measured as described above, whereas Rb isotope dilution analyses were done using the Zr-doping method [28] . Rb–Sr mica ages were derived by combining each phlogopite analysis with the Rb–Sr data for 77063L and R; calculations were done in ISOPLOT [29] . External precision (2 s.d.) for 87 Rb/ 86 Sr is 0.5%, and for 87 Sr/ 86 Sr is 0.01%. 87 Sr/ 86 Sr is reported relative to SRM987=0.710230. Rb–Sr model ages (±2 s.d.) for glauconite standard GLO-1 (89.3±0.8 Ma, n =16 over 7 years, assumed initial 87 Sr/ 86 Sr 0.7074) and SRM607 feldspar (1424±7 Ma, n =11 over 7 years, assumed initial 87 Sr/ 86 Sr 0.705) obtained using the same spike and techniques as those used for the phlogopites are consistent with Ar-Ar reference ages. Biotite GA1550 from Mount Dromedary (SE Australia) yields a Rb–Sr isochron age of 98.0±0.3 Ma ( n =9, 0.70445±6, MSWD (mean square weighted deviation) 1.6), consistent with Ar–Ar ages of 98.5±0.8 Ma [32] and 98.8±0.5 Ma [33] . Results are given in Table 4 . Semiquantitative trace element data for leachate–residue pairs (see above) indicate that most of the Hf resides in the residue (>90%), whereas Lu favours the leachates, consistent with their mineralogy and Bizimis et al. [34] . Overall, Lu–Hf budgets are dominated by the residue. Lu–Hf isotope analyses were therefore done on unleached whole rock powders. After dissolution at high pressure, a ~90% split of the solutions was spiked with a 176 Lu– 180 Hf tracer. Lu and Hf were isolated using a single-column technique [35] and measured by Multi-Collector-ICP-MS. The smaller split was equilibrated with a 233 U– 205 Pb tracer, followed by extraction of Pb and U on small columns of AG1-X8 (100–200 mesh, HBr-HCl) and EICHROM TRU resin (100–150 μm), respectively. Pb and U isotope ratios were measured by MC-ICP-MS [25] . Isotope dilution calculations for U–Pb were done with the EarthTime Excel U–Pb data reduction module [36] . 176 Hf/ 177 Hf was normalized to 179 Hf/ 177 Hf=0.7325 and reported relative to JMC475=0.282160. Internal precision (2se) for 176 Hf/ 177 Hf is ≤±0.000008, external precision ±0.000015 (2 s.d.). External precision for 176 Lu/ 177 Hf is ±1%. USGS standards BCR-2 and BHVO-2, analysed together with the kimberlite samples, yielded the following results: BCR-2, 0.50 ppm Lu, 4.94 ppm, 176 Lu/ 177 Hf 0.01439, 176 Hf/ 177 Hf 0.282868, 0.282875 and 0.282883; BHVO-2, 0.274 ppm Lu, 4.45 ppm Hf, 176 Lu/ 177 Hf 0.00877 and 176 Hf/ 177 Hf 0.283104. Modern CHUR has 176 Lu/ 177 Hf = 0.0332 and 176 Hf/ 177 Hf = 0.282772. The decay constant for 176 Lu is 1.865 10 −11 /year. Mass bias during U and Pb runs was corrected using internal normalisation to the natural U ratio and standard bracketing, respectively. External precision for 238 U/ 204 Pb is ±1% (2 s.d.). 232 Th/ 204 Pb was derived from 238 U/ 204 Pb measured by isotope dilution and Th/U from quadrupole ICP-MS trace element data on different splits of the same powders; expected errors ±10%. External precision for Pb isotope data is ≈±0.1−0.2% (2s.d. ); data reported are corrected for mass bias and blank (20±10 pg Pb). Uncertainties for calculated initial Pb isotope ratios, obtained by Monte Carlo simulation with the stated analytical uncertainties and an assumed age uncertainty of ±5 Ma: 206 Pb/ 204 Pb ±0.02, 207 Pb/ 204 Pb ±0.01, 208 Pb/ 204 Pb ≤±0.17. The decay constants are: 238 U 0.155125 × 10 −9 /year, 235 U 0.98485 × 10 −9 /year and 232 Th 0.049485 × 10 −9 /year. Lu-Hf and U-Pb isotope results are given in Table 5 . U–Pb LA-ICP-MS dating of perovskite U–Pb dating work on perovskite was performed during two analytical sessions: the first was done on polished grains in situ in blocks of fresh kimberlite samples 77063, 77081 and 77082; the second analytical session on the sample 77063 was performed on separated perovskite grains mounted in an epoxy block. The U–Pb analyses were performed at Macquarie University using a NewWave UP-213 laser ablation microprobe attached to an Agilent 7700 ICP-MS. The analytical technique was described in ref. 37 . Ablation occurs in He, permitting efficient sample transport, signal stability and reproducibility of U/Pb fractionation. The spot size varied between 30 μm for perovskite from the polished blocks and 40 μm for separated grains. Because of the smaller spot sizes used on the grains from the polished blocks, the analytical uncertainties are much higher for these grains. Samples were analysed in runs of 16 analyses comprising 12 analyses of unknowns bracketed by two analyses of a standard zircon (GEMOC GJ1, age 609 Ma) at the beginning and end of each run. The ‘unknowns’ include two near-concordant reference zircons, 91500 (ref. 38 ) and Mud Tank [39] , which are analysed before the samples and are used as independent control on reproducibility and instrument stability. The major problem of the U–Pb analysis of perovskite is the presence of high contents of common Pb. Instead of applying a common-Pb correction, we have used a regression technique, treating population of analyses from a single sample as representing mixtures between the common-Pb and radiogenic-Pb components. The intercepts of the regression line through the raw data on an inverse-Concordia (Tera-Wasserburg) plot thus provide both an estimate of the 207 Pb/ 206 Pb of the common-Pb component (upper intercept) and the inferred crystallization age (lower intercept). A total of 40 perovskites from sample 77063 were analysed during two sessions in April and June 2010. After rejection of 12 analyses with the largest analytical errors, the lower intercept of the regression line through the rest of the data ( n =28) gave an age of 113±13 Ma, which we consider as the best estimate for the crystallization age of this kimberlite ( Supplementary Fig. S1 ). Only 12 perovskites were found and analysed from sample 77081. These produce a high MSWD of 2.7 due to a scatter about the regression line. The rejection of four analyses had reduced this scatter (MSWD=0.63), giving the lower intercept age at 125±8 Ma and the best estimate for the crystallization age for this sample ( Supplementary Fig. S2 ). Sixteen out of 17 analyses done for sample 77082 produced a lower intercept age of 121±13 Ma, interpreted as crystallization age for this sample ( Supplementary Fig. S3 ). How to cite this article: Yaxley, G. M. et al. The discovery of kimberlites in Antarctica extends the vast Gondwanan Cretaceous province. Nat. Commun. 4:2921 doi: 10.1038/ncomms3921 (2013).